Transition from near-field thermal radiation to phonon heat conduction at sub-nanometre gaps When the separation of two surfaces approaches sub-nanometre scale, the boundary between the two most fundamental heat transfer modes, heat conduction by phonons and radiation by photons, is blurred. Here we develop an atomistic framework based on microscopic Maxwell’s equations and lattice dynamics to describe the convergence of these heat transfer modes and the transition from one to the other. For gaps >1 nm, the predicted conductance values are in excellent agreement with the continuum theory of fluctuating electrodynamics. However, for sub-nanometre gaps we find the conductance is enhanced up to four times compared with the continuum approach, while avoiding its prediction of divergent conductance at contact. Furthermore, low-frequency acoustic phonons tunnel through the vacuum gap by coupling to evanescent electric fields, providing additional channels for energy transfer and leading to the observed enhancement. When the two surfaces are in or near contact, acoustic phonons become dominant heat carriers. Heat conduction and thermal radiation are the two most fundamental modes of heat transfer. While thermal radiation heat exchange in the far field is limited to ∼ 6 W m −2 K −1 by Planck’s blackbody radiation law for two surfaces with temperatures close to 300 K, recent experiments [1] , [2] , [3] have shown that in the near-field when the two surfaces are separated by tens of nanometres the thermal conductance between two surfaces can increase by 3–4 orders of magnitude above the prediction by blackbody radiation, consistent with established theory based on fluctuating electrodynamics and macroscopic Maxwell equation [4] , [5] , [6] , [7] , [8] , [9] , [10] , [11] , [12] . In contrast, when two surfaces are in contact, heat transfer is described by conduction and for crystalline solids in terms of phonon transport [13] , and the thermal conductance values are in the range of 10 7 –10 9 W m −2 K −1 . Hence, 4–5 orders of magnitude increase in the thermal conductance are expected to occur as the two surfaces separation changes from tens of nanometres to contact. In the regime where the two surfaces are nearly in contact, there are no appropriate tools to describe the thermal transport process. This dilemma is analogous to recent strong interests in plasmon transport between two surfaces near contacts [14] , [15] , [16] , [17] , [18] especially when polar materials are used that support surface phonon polaritons similar to surface plasmons. In this paper, we develop an atomistic framework based on microscopic Maxwell’s equations and lattice dynamics to describe the convergence of these two modes of heat transfer and discuss the emerging physical picture of transition from near-field radiation to phonon heat conduction as two surfaces made of polar materials move from nanometre scale separation to contact. Continuum theory based on fluctuating electrodynamics and macroscopic Maxwell equations using bulk dielectric constant predicts d −2 dependence [2] , [16] of near-field radiation heat transfer between two surfaces supporting surface phonon polaritons in dielectric media and plasmons in metal media. As d approaches zero, the theory predicts that the heat transfer diverges. To address this issue, one approach is based on non-local dielectric constant in combination with macroscopic Maxwell equations [9] , [17] , [19] , [20] , [21] , [22] , [23] , [24] , [25] . In contrast, for heat conduction between two surfaces at contact, atomic Green’s function is often used to compute phonon transmission across interfaces [26] , [27] , [28] . Transport between polar materials for the case of small particles in close separation was studied using molecular dynamics simulation [29] and Green’s function [30] based on the van Beest, Kramer and van Santen (BKS) potential [31] that includes long-range static electromagnetic and short-range repulsive-attractive interactions. Reference [29] 29 established the equivalence between far-field radiation and dipole-dipole interaction at distances larger than the size of the particle and the dominance of closest atom-atom Coulomb interaction across the gap that smears near-field radiation and heat conduction. However, the trends at small spacing are difficult to interpret due to difficulties in shape and separation control of nanoparticles with the molecular dynamics technique in ref. 29 . Although acoustic phonon contribution was suggested in the study of silica clusters, the finite size of the nanoparticles makes the use of the language ‘phonon’ invalid [30] . Prunnila and Meltaus considered acoustic phonon tunnelling between piezoelectric materials in the electrostatic limit using a continuum description for the electric field and the strain in the material [32] . In this work, we present a unified atomic formalism combining microscopic Maxwell equations and atomic Green’s function to capture the physical picture of the transition from photon-mediated thermal radiation in the near-field to phonon-mediated heat conduction at contact. The formalism includes propagating electromagnetic waves and retardation effects. Taking into account the atomic details, this formalism does not need as input bulk/macroscopic properties such as a dielectric constant and inherently accounts for nonlocal effects. The formalism is applicable to thermal transport between any insulating objects with arbitrary separation including the far-field and contact limits. We apply this formalism to two semi-infinite bodies, which is a classical near-field radiative heat transfer problem first worked on on the basis of macroscopic fluctuating electrodynamics [5] . Our formalism resolves the divergence issue of the classical macroscopic theory but also reveals a higher conductance than its prediction as the two surfaces approach contact due to acoustic phonon tunnelling. Thus, this work provides insight about mechanisms of energy transfer in the transition from near-field thermal radiation to phonon heat conduction within a single unified formalism. Force constants We directly use the force interactions between atoms in the two bodies computed using microscopic Maxwell’s equations [33] as an input to a Green’s function formalism [27] to predict energy transmission. Unrestricted by the assumptions of the continuum theory, which smears out the atomic details, this approach is applicable at any gap. The approach is applied to NaCl because of the ready availability of harmonic force constants through the work of Jones and Fuchs [33] who computed the normal modes of vibration of NaCl using both short- and long-range interactions. This formalism is applicable to polar insulators where the electronic degrees of freedom are frozen. In the case of insulator–metal interfaces, one could extend the formalism to include the interaction with image charges in the metal to capture the coupling mechanism across the gap [34] , [35] . The short-range repulsive forces in sodium chloride arising due to the overlapping electron clouds of neighbouring ions are modelled here using the empirical nearest neighbour central potential developed by Kellerman [33] , [36] . These forces disappear across a gap and thus only play a role in connecting atoms within the bulk of the material (not across the gap). The long-range Coulomb forces are computed using the electric fields generated by oscillating ions; the exact expression for the long-range-retarded electric field E on any atom located at r , at time t , due to an oscillating atom at location r 0 , is provided below [33] , [37] , where q, ω, c and u are the charge, frequency of oscillation, speed of light and atomic displacement, respectively. The force due to the magnetic field, being on the order smaller, will be second order in the displacements, and is thus neglected in this formalism as was done in the work of Jones and Fuchs [33] . These long-range Coulomb forces exist at all length scales and are the only forces coupling atoms across a finite gap. The above microscopic approach correctly captures the behaviour of electromagnetic interactions for any separation between atoms ranging from few angstroms all the way to microns. This approach also exactly includes the effect of time retardation necessary for prediction of energy transfer at gaps of microns and larger. The rate of energy transfer through these force interactions across a gap is computed by using the atomistic Green’s function method [27] , [28] , [38] (see Methods for further details). This method yields the thermal conductance of a device (modelled here as two slabs of NaCl with a gap in between as a function of the interatomic spring constants). The electric forces in equation (1) are expanded to linear order in atomic displacements to define effective spring constants between atoms situated across the gap. Thus, this approach is ‘first-principles’ in the sense that the retarded Coulomb interactions between point charges across the gap, as well as the transmission function, are calculated exactly. It neglects anharmonicity and magnetic interactions, and is therefore valid at low temperatures and accurate up to correction terms. The formalism applies only to insulators, where conducting electrons do not exist. Thermal conductance According to the Landauer formalism [38] , [39] , we divide the system into three regions: the slabs of the ‘device’ region (a block of N layers split into two slabs, each N /2 layers) are sandwiched between semi-infinite left and right lead regions. These semi-infinite leads are represented by blocks, each block consisting of N atomic layers. The geometry is depicted in the inset in Fig. 1 . The long-range Coulomb forces were artificially truncated to only exist between adjacent blocks. To ensure that the long-range effects associated with Coulomb interactions were correctly included, the thickness of the blocks was progressively increased until the computed thermal conductance converged with respect to the layer thickness N to capture the limit of thermal conductance for two semi-infinite media. The accuracy of the force-constants was first checked by ensuring agreement between the computed phonon dispersion of a 7-layer slab with the results of Jones and Fuchs [33] . 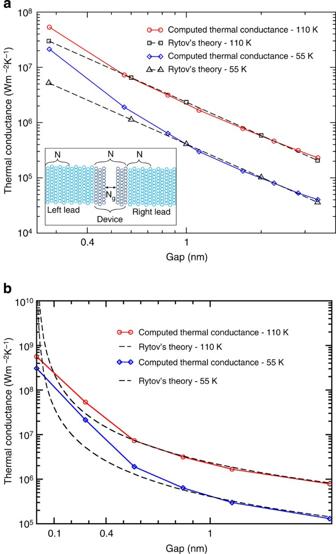Figure 1: Comparison of thermal conductance with continuum and atomic approaches. Computed thermal conductance at few nanometre gaps in (a) log-log and (b) semi-log at 110 and 55 K using atomistic formulations. The inset in (a) depicts a schematic of the system comprising semi-infinite leads and a central device region, divided into two slabs with a finite gap separating the surfaces. Figure 1: Comparison of thermal conductance with continuum and atomic approaches. Computed thermal conductance at few nanometre gaps in ( a ) log-log and ( b ) semi-log at 110 and 55 K using atomistic formulations. The inset in ( a ) depicts a schematic of the system comprising semi-infinite leads and a central device region, divided into two slabs with a finite gap separating the surfaces. Full size image The computed thermal conductance for gaps ranging from 0.3 to 2.8 nm is presented in Fig. 1a . At gaps >1 nm the thermal conductance computed using the atomistic approach agrees quantitatively with the spatially local continuum theory (based on Rytov’s formulation) that shows an inverse d 2 behaviour with gap size. In the continuum approach, the local dielectric constant, which is only a function of frequency, was derived through the same force interactions (using equation (8.2) in Jones and Fuchs [33] ) that we used in the atomic theory for computing thermal conductance through the Green’s function method (See Methods for more details), allowing consistency between the two methods and thus a direct comparison of the predicted thermal conductances. The agreement between the two methods at gaps >1 nm provides a validation of the atomistic method. Our approach avoids the divergence issue as d approaches zero that exists in the continuum theory ( Fig. 1b ). While nonlocal dielectric theory can resolve the issue of the divergence [9] , [17] , [19] , [20] , [21] , [22] , [23] , [24] , [25] , the atomic formalism presented here not only inherently accounts for nonlocal effects due to atomic considerations for the electromagnetic fields, but also has the virtue of accounting for the short-range bonding forces, which provide another channel for enhancement in thermal conductance and must be included for an accurate description of the interaction between the layers at sub-nanometre gaps. Interestingly, at gaps <1 nm and before contact, the atomistic approach predicts conductances significantly higher than the continuum approach. For example, at 55 K the predicted conductance is higher by 1.5 and 4 times at gaps of 0.56 and 0.28 nm, respectively (see Fig. 1 ). Here the contact limit (0 gap) is the case of bulk sodium chloride, that is, the spacing between the surface atoms is exactly the lattice spacing. Finite gaps are further separation from this bulk limit. At higher temperatures this enhancement diminishes in magnitude; at a temperature of 110 K the enhancement is by a factor of 1.8 at a gap of 0.28 nm. The large enhancement in heat transfer at sub-nanometre gaps points to a breakdown of the continuum approach at these length scales. A similar effect was observed in molecular dynamics simulation of heat transfer between two adjacent nanoparticles [29] . However, due to the nature of the molecular dynamics simulations that resulted in the change in structure of the nanoparticles, the gap dependence is difficult to justify for distances comparable to the particle size. The formalism used by Domingues et al . [29] includes electrostatic interactions via inter-atomic potential as is justified by the comparison made between the distance separating the nanoparticles and the wavelength. The interpretation of their results relies on the size of the particles. Our atomistic framework includes the full radiative time-retarded fields and can provide a more systematic understanding of the role time retardation can play at gaps for which the static limit assumption breaks down. Acoustic phonon tunnelling To explain the enhancement, we begin by looking at energy transmission functions as a function of frequency ( Fig. 2a–f ) and wavevector ( Fig. 2g–l ) for gaps ranging from 0 to 2.8 nm, where the atomic formalism and the continuum formalism are well converged. While at perfect contact heat transfer is classically due to thermal conduction and is dominated by low-frequency phonons ( Fig. 2a ), at gaps > 1 nm heat transfer is only by phonons with frequencies >200 cm −1 ( Fig. 2d–f ). Fig. 3a (computed phonon dispersion of bulk NaCl using the force interactions outlined earlier) shows that these high-frequency phonons are the optical phonons, being higher than the acoustic-optic crossing value of 140 cm −1 . This agrees well with the understanding of near-field photon tunnelling across gaps between polar dielectric materials through resonant coupling of electric fields with high-frequency optical phonons, that is, phonon-polaritons [1] , [3] , [4] , [8] , [9] , [40] , [41] . However, as the gap is decreased from 1 nm to 0.56 and 0.28 nm we find that in addition to optical phonons even low-frequency acoustic phonons begin to contribute to heat transfer ( Fig. 2b,c ). At a gap of 0.28 nm phonons with frequencies <140 cm −1 contribute almost 63% and 42% to total thermal conductance at 55 and 110 K, respectively. These phonons are mostly acoustic (see Fig. 3a ). This tunnelling of acoustic phonons through evanescent electric fields provides new channels for heat transfer at sub-nanometre gaps, blurring the distinction between conduction and radiation modes of heat transfer at these length scales. 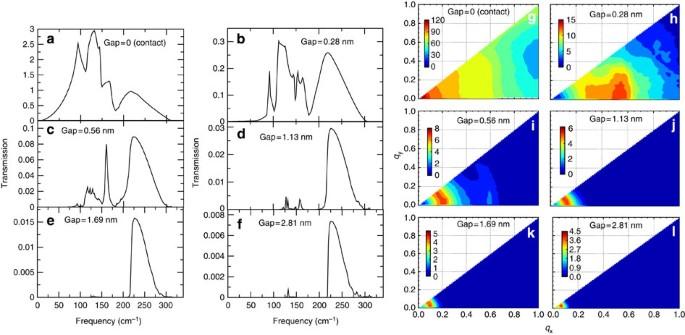Figure 2: Dependence of transmission function on gap spacing and wavevector. (a–f) Transmission integrated overqas a function of frequency. (g–l) Thermal conductance as a function of transverse wavevector, integrated over frequency, for different gaps of 0, 0.28, 0.56, 1.13, 1.69 and 2.81 nm. (In the contour plots the region close to the light cone cannot be seen as it is too small in magnitude, to give an estimate for the peak frequencyω∼320 cm−1,q∼ω/c∼0.01π/a). The wavevectors in the plots are normalized by the lattice constant usingπ/a, wherea=2.8 nm is the spacing between atomic layers in NaCl. Note the maximum in transmission scales as the inverse of the gap. Figure 2: Dependence of transmission function on gap spacing and wavevector. ( a – f ) Transmission integrated over q as a function of frequency. ( g – l ) Thermal conductance as a function of transverse wavevector, integrated over frequency, for different gaps of 0, 0.28, 0.56, 1.13, 1.69 and 2.81 nm. (In the contour plots the region close to the light cone cannot be seen as it is too small in magnitude, to give an estimate for the peak frequency ω ∼ 320 cm −1 , q ∼ ω / c ∼ 0.01 π / a ). The wavevectors in the plots are normalized by the lattice constant using π / a , where a =2.8 nm is the spacing between atomic layers in NaCl. Note the maximum in transmission scales as the inverse of the gap. 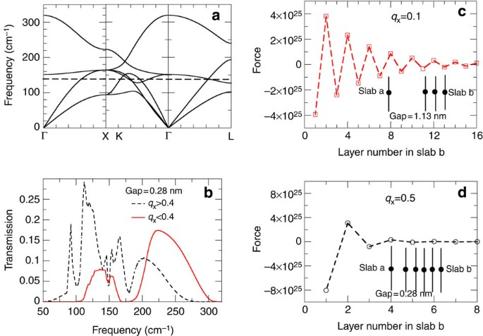Figure 3: Effects of large and small wavevector. (a) Computed phonon dispersion of bulk NaCl. (b) Transmission at a gap of 0.28 nm due to large and small wavevectors. (c) Force on a surface atom in slab a due to atoms in slab b in different layers for gap of 1.13 nm forqx=0.1 andqy=0.05. (d) Same force for a gap of 0.28 nm forqx=0.5 andqy=0.1. The insets of (c) and (d) depict an atom (dot) in the surface layer (line) of slab ‘a’ interacting with atoms in various layers of slab ‘b’. Full size image Figure 3: Effects of large and small wavevector. ( a ) Computed phonon dispersion of bulk NaCl. ( b ) Transmission at a gap of 0.28 nm due to large and small wavevectors. ( c ) Force on a surface atom in slab a due to atoms in slab b in different layers for gap of 1.13 nm for q x =0.1 and q y =0.05. ( d ) Same force for a gap of 0.28 nm for q x =0.5 and q y =0.1. The insets of ( c ) and ( d ) depict an atom (dot) in the surface layer (line) of slab ‘a’ interacting with atoms in various layers of slab ‘b’. Full size image Such a tunnelling effect involving acoustic phonons can be understood by looking at the dependence of thermal conductance on transverse vibration wavevectors q (parallel to the slabs) involved. At perfect contact of zero gap all wavevectors participate and thermal transport can be explained by classical thermal conduction where large wavelength acoustic phonons dominate ( Fig. 2g ) At gaps >1 nm only the small wavevectors ( q ) contribute to thermal conductance (see Fig. 2j–l ). These differences in the magnitude of the wavevectors involved at different length scales are related to the decay length of the generated evanescent electric fields. Electric fields vary with wavevector q and spacing d as e −( qd ) ; at large gaps (large d ) only the fields that decay slowly with distance couple the two slabs; these are the small q electric fields and play the dominant role in heat transfer at large gaps (It should be noted that very small wavevectors q close to the light cone also couple slabs at all gaps; however, force constants coupling the slabs are proportional to qe −( qd ) . This behaviour can be explained by noting that the 2D Fourier transform of the Coulomb potential in real space , where d is the gap spacing and r is the distance in the 2D crystal plane, yields in Fourier space , and since the force constants are the second derivative of the potential, their dependence is proportional to qe −( qd ) . For very small these forces are too weak to play any role at gaps smaller than micrometres and hence their contribution to thermal conductance for nanoscale gaps is negligible). The optimal wavevector that maximizes these force constants varies like . This explains why as the gap is increased, the dominant contribution to the heat transfer shifts to smaller q to optimize the force qe −( qd ) but is not exactly zero. The contour plots reflect that the dominant contribution for a gap is at a finite value and not at the q =0 point ( Fig. 2j–l also confirm the 1/ d dependence). Therefore, the dominant wavevectors for which transmission is largest, even though small, are well outside of the light cone. In this sense, for these sub-nanometre gaps, the limit may be taken and the retarded nature of forces will not be relevant in the region of large transmission for these sub-nanometre gaps. Figure 3b shows that heat transfer by high frequency optical phonons is driven mostly by these small q fields. These slowly decaying electric fields ( ∼ e −( qd ) ) lead to force interactions that span several tens of layers in either slab (see Fig. 3c that shows these forces between an atom in slab ‘a’ and atoms in slab ‘b’). Opposite polarity of ions in the adjacent layers leads to such forces being highly oscillatory; these forces then couple in a resonant manner with high-frequency optical phonons (involving out of phase vibration of adjacent ions). Such force interactions, which involve tens of layers of either slab, are adequately captured by a bulk local dielectric constant and lead to the success of the continuum approach. However, as gaps are decreased to sub-nanometre lengths, we find that additional large wavevector ( q ) fields (see Fig. 2h,i ), which decay rapidly with spacing and hence are only able to lead to force interactions at these very small gaps (approaching atomic spacing), also come into play. Figure 3b shows that heat transfer by the low-frequency acoustic phonons (discussed earlier) is mostly driven by these large q electric fields. At large q (see Fig. 3d ) the rapidly decaying fields are only able to cause force interactions between 1 or 2 surface layers of either of the two slabs across the gap. These forces do not have a strong oscillatory nature across multiple layers; instead, these surface–surface interactions rather resemble the short-range forces due to overlapping electron clouds [36] that only exist between neighbouring ions. These ‘short-range’ Coulomb interactions across the gap combine with both short-range and long-range interactions within the bulk lead to transmission through both collective vibration of atoms (acoustic phonons) as well as optical phonons. Such surface–surface interactions at sub-nanometre gaps cannot be accurately captured by a bulk dielectric constant. They require a non-local wavevector-dependent description and lead to the observed enhancement in thermal conductance above that predicted by continuum theory based on macroscopic Maxwell equations. The breakdown of the local dielectric approach here occurs over a length scale comparable to the lattice constant. Previous studies similarly reported results on the breakdown of the local dielectric approach in predicting the absorption properties of magnesium oxide nanoparticles [42] . In the case of nanoparticles, the size dependence was shown for a surface mode in the optical phonon frequency range [42] , while our approach shows that the enhancement to thermal transport in the sub-nanometre range due to the unscreened interaction between the surface layers (see Fig. 3d ) involves both acoustic and optical phonons at gaps comparable to the lattice constant (see Fig. 2b,c ). The different enhancement magnitudes at 55 and 110 K can be understood by noticing that, at 55 K, the high-energy optical phonons that drive conductance at larger gaps are not well populated. As the gap is reduced to 0.28 nm low-energy acoustic phonons come into play, these are relatively more populated and lead to sharp increase in conductance. At a higher temperature of 110 K, however, even the high-energy phonons are relatively more excited, and the addition of acoustic phonons leads to only a moderate increase in conductance. It should be noted that while such an acoustic phonon tunnelling was presented in a continuum formalism by Prunnila et al. [32] where the coupling between phonons and the electromagnetic field was due to the piezoelectric effect, our work reveals that such tunnelling effects can exist at sub-nanometre length scales even in bulk systems without any piezoelectric effects. The tunnelling of acoustic phonons across a vacuum finite gap was previously suggested based on nonequilibrium interaction of an STM tip with a metal substrate [34] . For interacting metal surfaces, the electromagnetic field provided the coupling mechanism between electrons and phonons. It should also be noted that the effect presented in this letter, of enhancement in heat transfer through tunnelling of acoustic phonons, is in addition to the effect of enhancement in conductance due to overlapping electron clouds observed by Xiong et al. [30] for the case of interacting finite-sized nanoparticles. Although the importance of low frequency vibrations was verified for small gaps in ref. 30 , the small cluster size excludes long-wavelength acoustic phonons and leads to (particle-)size dependence of near-field radiation heat transfer in addition to gap dependence, as is evident in the observation of heat transfer versus gap changing from d −12 , to d −3 , to d −2 , while our simulation shows agreement with classical fluctuating electrodynamics prediction of d −2 when d becomes > ∼ 1 nm. A recent work also considered the enhancement of thermal transport due to the acoustic phonons and utilized the language of ‘induced phonon transfer’ to account for the transmission of acoustic phonons in one material due to the electromagnetic coupling with another [43] . The work highlighted the importance of the acoustic phonon transfer as a dominant mechanism at small gaps comparable to the lattice constant but only considered a local dielectric constant in considering the electromagnetic interaction between the surfaces. The authors duly noted the importance of a more sophisticated approach as presented here for understanding the transition from radiation to conduction. In summary we have developed an atomistic framework based on microscopic Maxwell’s equations and lattice dynamics to describe the transition from near-field radiation to heat conduction when two surfaces are close to contact. Predicted conductances agree well with the continuum approach at gaps >1 nm validating this atomistic framework; however, at sub-nanometre gaps the two approaches differ significantly with the atomistic approach predicting an almost four times increase in conductance compared with the continuum approach, while avoiding the divergence dilemma at contact in the continuum approach. This suggests that at gaps approaching the spacing between the atomic layers the continuum approach based on local bulk dielectric constant breaks down. In addition, the present theory provides insight about the physical nature of energy transfer at the nanoscale. Owing to the presence of the vacuum gap, at large gaps, the far-field energy transfer is through photons. As the gap becomes smaller, the mediation shifts to surface polaritons in the near-field regime, followed by acoustic phonon tunnelling at sub-nanometre gaps and finally, at contact, to phonon transmission or conduction. All these regimes are captured within a single formalism, demonstrating a complete picture of the transition of radiation to conduction. This approach is important for understanding thermal interface resistance and can be extended so that each side is made of different materials. These results are useful for accurate modelling of technologies such as heat-assisted magnetic recording [44] , thermal contact resistance between different materials [26] , [45] , thermal conductivity of porous materials such as aerogels [46] where the gaps demonstrated are on the nanometre and sub-nanometre length scales. Atomic Green’s function formalism The nonequilibrium atomic Green’s function formalism is a method used to calculate thermal transport through a material, which is divided into a ‘device’ region, sandwiched between hot and cold thermal reservoirs represented by semi-infinite leads (see refs 27 , 39 for detailed description and procedure). It takes as input the force constants derived from the interactions between the atoms in the harmonic limit and calculates the transport of energy from the hot reservoir to the cold reservoir. The transmission Tr obtained from the Green’s function approach is and we note that each term depends on the transverse momentum q and incident phonon frequency ω (refs 27 , 28 , 39 ). The dependence on the transverse momentum q arises due to the transverse Fourier transform exploiting periodicity in the transverse directions to decouple the 3D system to a sum of 1D chains for each transverse momentum [43] . The retarded Green’s function of each 1D chain can be deduced from G s =[( ω + i Δ) 2 I – H d –Σ L –Σ R ] −1 where Δ is an infinitesimal part that maintains the causality of the Green’s function and Σ L and Σ R are the self energies of the left and right leads with and . The dynamics of the lead atoms is calculated as a functional of the device atoms, so the self energies are the result of projecting the interactions between the device and lead regions onto the device region [39] . The Lopez-Sancho algorithm [47] , [48] is used to efficiently numerically calculate the projection of the leads onto the device region. H d is the force constant matrix of the device region [27] derived using both the short-range and the long -ange Coulomb interactions discussed above. In this Green’s function approach, force interactions are taken to exist only between neighbouring blocks and between the device and adjacent block, and the size of the blocks is systematically increased to ensure convergence to the semi-infinite system. Local dielectric constant The dielectric constant is calculated from the lattice dynamics of the atomic system subjected to an external electric field utilizing Equation (8.2) of the work of Fuchs et al. [33] The results of the real part are fitted to the Drude–Lorentz model, and the imaginary part is constructed utilizing the Kramers–Krong relations to obtain an analytic form for the dielectric constant. This is then used in the fluctuation dissipation theorem to calculate transport in the fluctuating electrodynamics formalism [5] , [6] . The interactions used to calculate the local dielectric constant are the same as those input into the Green’s function formalism allowing for an appropriate comparison between the two models for large gaps. How to cite this article: Chiloyan, V. et al. Transition from near-field thermal radiation to phonon heat conduction at sub-nanometre gaps. Nat. Commun. 6:6755 doi: 10.1038/ncomms7755 (2015).